Ferroelectrically driven spatial carrier density modulation in graphene The next technological leap forward will be enabled by new materials and inventive means of manipulating them. Among the array of candidate materials, graphene has garnered much attention; however, due to the absence of a semiconducting gap, the realization of graphene-based devices often requires complex processing and design. Spatially controlled local potentials, for example, achieved through lithographically defined split-gate configurations, present a possible route to take advantage of this exciting two-dimensional material. Here we demonstrate carrier density modulation in graphene through coupling to an adjacent ferroelectric polarization to create spatially defined potential steps at 180°-domain walls rather than fabrication of local gate electrodes. Periodic arrays of p – i junctions are demonstrated in air (gate tunable to p – n junctions) and density functional theory reveals that the origin of the potential steps is a complex interplay between polarization, chemistry, and defect structures in the graphene/ferroelectric couple. The extraordinary properties of chiral Dirac fermions make graphene a promising platform to harness relativistic, two-dimensional phenomena for a wide range of electronic and optoelectronic applications [1] , [2] , [3] . Exploitation of these effects, however, requires local control over the charge carrier density in graphene. The creation of spatially defined p – n junctions in graphene is of critical importance for the modulation of chiral tunnelling [3] , [4] , magnetoresistance [5] , electron beam collimation [6] , Veselago lensing [7] and terahertz plasmonic devices [8] . Arrayed junctions have been predicted to give anisotropic group velocity renormalization of charge carriers and new Dirac points [9] , [10] , [11] , and could also open a transmission gap [12] , increasing the typically low on/off ratios in graphene transistors. The deterministic implementation and widespread use of these promising phenomena, however, is limited by the necessity for multiple gate electrodes, complex fabrication and electrical wiring and added power consumption. A low-power, simple alternative to complex split-gate electrodes can be achieved by coupling graphene to an adjacent, remanent ferroelectric polarization, which can drive changes in the graphene via electrostatic doping from interaction with the polarization [13] . Devices based on this concept have demonstrated non-volatile resistance hysteresis [13] , [14] , [15] and transparent conductivity in flexible electronics [16] , [17] . Initial experimental studies, however, achieved charge density changes in graphene much smaller than anticipated from full compensation of the polarization [18] , since the electrostatic coupling can be limited by extrinsic effects caused by adsorbed molecules [15] , [19] , [20] . The atomistic details and interfacial chemistry governing the interaction and the resulting charge density changes in graphene remain elusive. In addition, polydomain ferroelectrics and their interactions with graphene have received limited theoretical and experimental attention. Here, we provide a comprehensive understanding of the coupling between the graphene doping level and ferroelectric polarization, including local manipulation of carrier density and type in graphene, and atomistic and electronic details of the interface. Experimental observations of charge density modulation in graphene/LiNbO 3 couples qualitatively match the intuitive picture of compensation of the ferroelectric polarization that should lead to n - or p -doping for ferroelectric polarization pointing towards or away from graphene, respectively. First-principles density functional theory (DFT) calculations, however, reveal that this seemingly simple coupling is highly dependent on the net surface-bound charge of the ferroelectric. To simulate the experimental observations, we include in the model all the intrinsic influences on the interfacial chemistry, including the polar stacking, ferroelectric polarization, surface reconstruction, and sample history, yielding an upper limit for the expected carrier density modulation. We propose chemical mechanisms based on the extrinsic effects from defects induced by the transfer process to explain the reduction in the observed charge density modulation. Armed with this knowledge, we demonstrate the versatility provided by leveraging such coupling, including the use of alternating carrier density/type in graphene on periodically poled ferroelectrics for the formation of p – i , p – n , or n – i junctions. This graphene/ferroelectric interface also offers a novel and straightforward route for the creation of periodic potentials in graphene through spatially deterministic control over charge carriers without the need for complex local gates. Ferroelectricity-induced carrier density modulation Graphene sheets grown via chemical vapour deposition were transferred to commercially available periodically poled and single-domain LiNbO 3 substrates (Asylum Research), using an established wet transfer process [15] . High-resolution Raman spectroscopy [21] was used to probe the graphene/LiNbO 3 structures and map the domain structure of the LiNbO 3 by measuring the shift in the frequency of the E (TO8) band that occurs near domain boundaries [22] , [23] ( Fig. 1a ). A piezoresponse force microscopy image acquired prior to graphene transfer verified the same 10-μm periodicity of up- and down-polarized domains as the Raman image ( Fig. 1a , inset). On the basis of the intuitive picture described previously [15] , [19] , [20] , we expect the Kronig–Penney-type potential landscape exhibited by this domain configuration to create a spatially periodic charge carrier density modulation in the graphene, with increased and decreased electron concentrations in graphene in contact with up- and down-polarized domains, respectively. Shifts in the Raman G-band mode frequency [24] , [25] , [26] provide a spatially resolved probe of the carrier density in graphene without the need for device fabrication, which could screen or alter the nature of the interactions [27] , [28] ( Fig. 1b ). Raman G-band frequency mapping revealed that periodic regimes of lower and higher frequency indeed correlate directly to up- and down-polarized domains, respectively. These periodic shifts from lower to higher Raman frequency correspond to sharp transitions at the ferroelectric domain walls between low and high carrier concentrations in the graphene (this is further confirmed by observation of changes in the graphene two-dimensional-band frequency and intensity, Supplementary Fig. 1 ). Domain walls in ferroelectrics are generally 0.5–10 nm wide [29] and thus provide a novel and promising route to achieve deterministic and precise spatial control over the carrier density in graphene that is comparable to the intrinsic depletion width expected in graphene [30] . 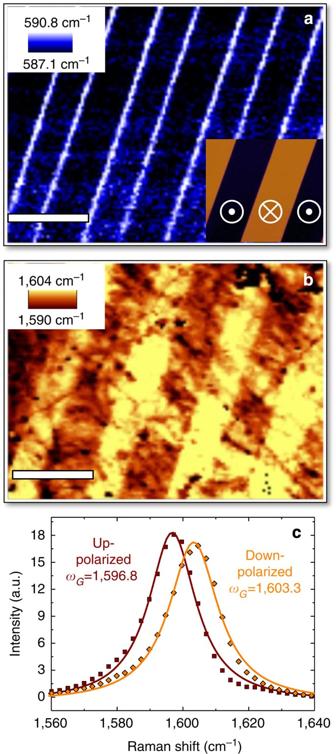Figure 1:Raman spectroscopy of graphene/LiNbO3heterostructures. (a) LiNbO3E(TO8) frequency map. The inset shows a corresponding PFM phase image of the same LiNbO3sample before graphene transfer. (b) Graphene G-band frequency map. Spectra were collected simultaneously to the map ina. Scale bars, 10 μm. (c) Graphene G-peak averaged over a dark and a bright stripe inbwith the G-band frequencyωG=1,603.3 cm−1and 1,596.8 cm−1for bright and dark stripes, respectively. Lines correspond to Lorentzian fits to the experimental data (orange diamonds for the bright stripe and dark-red squares for the dark stripe). Figure 1: Raman spectroscopy of graphene/LiNbO 3 heterostructures. ( a ) LiNbO 3 E (TO8) frequency map. The inset shows a corresponding PFM phase image of the same LiNbO 3 sample before graphene transfer. ( b ) Graphene G-band frequency map. Spectra were collected simultaneously to the map in a . Scale bars, 10 μm. ( c ) Graphene G-peak averaged over a dark and a bright stripe in b with the G-band frequency ω G =1,603.3 cm −1 and 1,596.8 cm −1 for bright and dark stripes, respectively. Lines correspond to Lorentzian fits to the experimental data (orange diamonds for the bright stripe and dark-red squares for the dark stripe). Full size image More quantitative information about the carrier concentration and type in the graphene/ferroelectric hybrid structures was obtained by comparing the average Raman G-band frequency measured for graphene on up- and down-polarized domains ( Fig. 1c ). The peak positions for graphene on up- and down-polarized domains were 1,597 and 1,603 cm −1 , respectively, corresponding to a carrier density difference of ~4 × 10 12 cm −2 , assuming both stripes are p -doped [24] , which is typical for graphene on ferroelectrics in air [15] . The doping level in the different domains can be further quantified and the carrier type unambiguously extracted if a gate potential is applied. For this purpose, top-gated graphene transistors on single-domain and periodically poled LiNbO 3 were fabricated employing an electrolyte top gate (LiClO 4 in a poly(ethylene oxide) medium) [31] ( Fig. 2a,b ). The representative gate-voltage-dependent Raman G-band shift on a single-domain, down-polarized sample reveals p -doped behaviour, while a similar device on an up-polarized sample is nearly intrinsic ( Fig. 2c ). The corresponding gate-dependent conductance independently verifies p -doping on down-polarized LiNbO 3 and nearly intrinsic graphene on up-polarized LiNbO 3 (inset, Fig. 2c ). The characteristics shown here are representative of the Dirac points observed for 10 devices fabricated for each polarity. Using the same top-gating procedure on a device fabricated on a periodically poled LiNbO 3 substrate, the gate dependence of the regimes of lower and higher Raman frequency ( Fig. 1b ) can be used to gain further insight into the actual doping level and carrier type of graphene. The same Raman trend observed for devices on single-domain LiNbO 3 is observed for the corresponding stripes (that is, graphene is p -type on down-polarized domains and nearly intrinsic on up-polarized domains) ( Fig. 2d ). The actual carrier density can be estimated using the quantum capacitance of the graphene channel and the geometrical gate capacitance [24] , [31] , resulting in a carrier density difference of ~3 × 10 12 cm −2 , further supporting the observations based on the Raman frequencies ( Fig. 1c ). Considering the spatial control over the doping level through the ferroelectric domain structure and the observed carrier density differences, the periodic modulation ( Fig. 1b ) corresponds to a graphene sheet with multiple, parallel p – i junctions. This proof of concept could potentially be combined with advances in nanoscale domain engineering in ferroelectrics [32] , [33] or deterministic patterning [34] to create such periodic arrays with periodicities many orders of magnitude smaller than those demonstrated here, which could be particularly impactful for inducing and studying exotic phenomena in graphene. 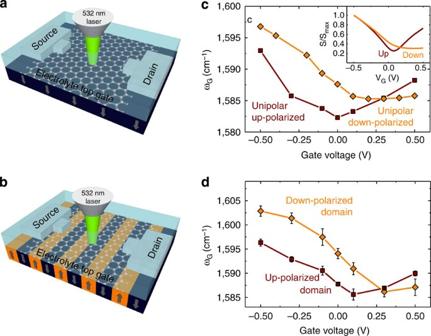Figure 2:Gate-dependent Raman spectroscopy of graphene on unipolar and periodically poled LiNbO3. Schematic of a top-gated graphene transistor on (a) unipolar and (b) periodically poled LiNbO3. (c) Representative gate-dependent Raman G-band frequency for a single-domain, down-polarized (orange diamonds) and a single-domain, up-polarized (dark-red squares) device. (d) Representative gate-dependent Raman G-band frequency averaged over a down-polarized domain (orange diamonds) and an up-polarized domain (dark-red squares). Error bars indicate the s.d. of the frequency within each stripe. Figure 2: Gate-dependent Raman spectroscopy of graphene on unipolar and periodically poled LiNbO 3 . Schematic of a top-gated graphene transistor on ( a ) unipolar and ( b ) periodically poled LiNbO 3 . ( c ) Representative gate-dependent Raman G-band frequency for a single-domain, down-polarized (orange diamonds) and a single-domain, up-polarized (dark-red squares) device. ( d ) Representative gate-dependent Raman G-band frequency averaged over a down-polarized domain (orange diamonds) and an up-polarized domain (dark-red squares). Error bars indicate the s.d. of the frequency within each stripe. Full size image Interfacial chemistry of graphene/ferroelectric couples While the observed carrier density difference in graphene on periodically poled LiNbO 3 is in accordance with previous results [15] , it is two orders of magnitude lower than the value expected from full compensation of the bulk ferroelectric polarization. A more complete exploration of the graphene/LiNbO 3 interface considering the interfacial chemistry effects from the exposed experimental environment is therefore imperative. To investigate the nature of the interaction of graphene and the ferroelectric polarization, we employed first-principles DFT calculations on a model system consisting of a single-domain ferroelectric LiNbO 3 (0001) slab with graphene sheets on both the up-polarized ( P + , polarization pointing towards the graphene) and the down-polarized ( P − , polarization pointing away from the graphene) surfaces. A number of possible graphene/ferroelectric interfacial configurations were explored (details in Supplementary Fig. 2 ). All configurations suggest that the interaction at the graphene/ferroelectric interface is driven by physisorption. To understand the electronic structure of the interface, the net surface charges in the LiNbO 3 are of the utmost importance. For paraelectric LiNbO 3 (0001), the polar stacking, consisting of equally spaced LiO 3 (−5 e ) and Nb (+5 e ) layers, leads to surface charges of −5 e /2 and +5 e /2 per surface unit cell for the stoichiometric LiO 3 and Nb terminations, respectively. The bulk ferroelectric polarization at 0 K is P 0 ≈0.86 C m −2 (as computed with the Berry’s phase approach), and this reduces the net bound charge to −1.34 e and 1.34 e per surface cell in the LiO 3 - ( P + ) and Nb-terminated ( P − ) surfaces, respectively. These surface charges must be passivated by mobile charges, surface reconstructions and/or, in this case, the graphene. It has been demonstrated that the most thermodynamically favourable surface charge passivation mechanism in ferroelectric LiNbO 3 is by surface chemical reconstructions [35] , where additional Li ions on the P + surface and additional O and Li on the P − surface reduce the net surface charge [35] , [36] . Taking into account the strong impact of the inherent polarity, surface reconstructions and temperature-dependent ferroelectric polarization, P ( T ), on the resulting net surface charge, we probed the evolution of the LiNbO 3 surface under realistic sample history. Experimentally, the LiNbO 3 sample was annealed at 473 K to reduce defects induced by the poling process and was then cooled down to room temperature, 298 K, in air prior to the transfer of the single-layer graphene to the surface in water. Simulating such a scenario where the polarization is allowed to vary with temperature and assuming a 2 × 1 surface unit cell of LiNbO 3 with three extra Li ions per P + and three extra Li–O per P − surface cell ( Fig. 3a–c ) allowed us to develop a more representative model of the actual device. During the annealing process, there is a threshold temperature above which surface reconstruction occurs to achieve the most stable configuration and minimization of the net surface charge, but upon transitioning below that threshold temperature it is no longer kinetically possible to further change the surface stoichiometry. Using a Landau model ( Supplementary Fig. 3 ), we can calculate the bulk P ( T ). The P (473 K)=0.8 P 0 and, assuming that the threshold temperature is the same as the annealing temperature of 473 K (representing the maximum effect possible), the surface is allowed to reconstruct to address the need to compensate the polarization in LiNbO 3 . If experimental limitations allowed the deposition of graphene to these fully compensated surfaces at the high-temperature reconstruction (and T =473 K), our model finds that graphene on both the P + and P − surfaces would be intrinsic ( Fig. 3d ). In other words, compensation is achieved by the LiNbO 3 itself, and the graphene provides no additional compensation. 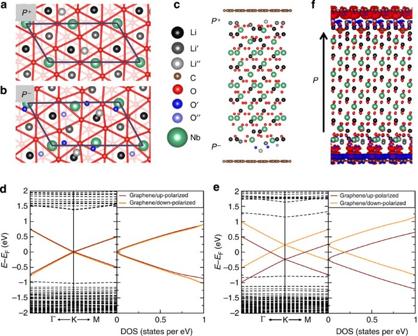Figure 3:Atomic and electronic structure of the graphene/LiNbO3(0001) interface. Relaxed atomic surface structures of LiNbO3with graphene (not shown for clarity) adsorbed on the (a) up-polarizedP+surface (with a 2 × 1 nonstoichiometric reconstruction with an extra Li, denoted as Li', per surface unit cell and an extra Li, denoted as Li'', per every two surface unit cells) and (b) down-polarizedP−surface (with a 2 × 1 nonstoichiometric reconstruction with an extra Li–O, denoted as Li' and O', per surface unit cell and an extra Li-O, denoted as Li'' and O'', per every two surface unit cells). The dark-purple line indicates the surface lattice periodicity. (c) Atomic structure of the 2 × 1 surface reconstructed slab with graphene adsorbed on both terminations, reconstructed adatoms and two trilayers (Li–O3–Nb) near each interface are allowed to relax while the rest of the film, in this case, is fixed to theP(298 K)=0.875P0atomic positions. Colour-coded labels indicate the ions that substantially passivate the polarization surface charge in the surface reconstruction. (d) Electronic band structure of graphene on both up- and down-polarized ferroelectric surfaces demonstrating that graphene is intrinsic for both interfaces in a relaxed slab with internal bulk ferroelectric polarization fixed toP(473 K)=0.8P0, where the surface charge is essentially fully passivated by the 2 × 1 reconstruction. (e) Induced charge redistribution as the graphene/ferroelectric interfaces are formed, where red indicates the gain of electrons (up-polarized, top surface) and blue the gain of holes (down-polarized, bottom surface), for the hybrid structure shown inb. The isovalue used to plot the charge density differential is 0.002eÅ−3. (f) Electronic band structure of graphene on both up- and down-polarized ferroelectric surfaces demonstrating that graphene becomesn-doped andp-doped, respectively, passivating the extra surface charge that emerges in the 2 × 1 reconstructed surfaces as temperature is reduced from 473 to 298 K and the ferroelectric polarization increases fromP(473 K)=0.8P0toP(298 K)=0.875P0. Figure 3: Atomic and electronic structure of the graphene/LiNbO 3 (0001) interface. Relaxed atomic surface structures of LiNbO 3 with graphene (not shown for clarity) adsorbed on the ( a ) up-polarized P + surface (with a 2 × 1 nonstoichiometric reconstruction with an extra Li, denoted as Li', per surface unit cell and an extra Li, denoted as Li'', per every two surface unit cells) and ( b ) down-polarized P − surface (with a 2 × 1 nonstoichiometric reconstruction with an extra Li–O, denoted as Li' and O', per surface unit cell and an extra Li-O, denoted as Li'' and O'', per every two surface unit cells). The dark-purple line indicates the surface lattice periodicity. ( c ) Atomic structure of the 2 × 1 surface reconstructed slab with graphene adsorbed on both terminations, reconstructed adatoms and two trilayers (Li–O 3 –Nb) near each interface are allowed to relax while the rest of the film, in this case, is fixed to the P (298 K)=0.875 P 0 atomic positions. Colour-coded labels indicate the ions that substantially passivate the polarization surface charge in the surface reconstruction. ( d ) Electronic band structure of graphene on both up- and down-polarized ferroelectric surfaces demonstrating that graphene is intrinsic for both interfaces in a relaxed slab with internal bulk ferroelectric polarization fixed to P (473 K)=0.8 P 0 , where the surface charge is essentially fully passivated by the 2 × 1 reconstruction. ( e ) Induced charge redistribution as the graphene/ferroelectric interfaces are formed, where red indicates the gain of electrons (up-polarized, top surface) and blue the gain of holes (down-polarized, bottom surface), for the hybrid structure shown in b . The isovalue used to plot the charge density differential is 0.002 e Å −3 . ( f ) Electronic band structure of graphene on both up- and down-polarized ferroelectric surfaces demonstrating that graphene becomes n -doped and p -doped, respectively, passivating the extra surface charge that emerges in the 2 × 1 reconstructed surfaces as temperature is reduced from 473 to 298 K and the ferroelectric polarization increases from P (473 K)=0.8 P 0 to P (298 K)=0.875 P 0 . Full size image Upon cooling the LiNbO 3 , however, the polarization of the ferroelectric will increase, and unpassivated surface charge resulting directly from the increase in bulk ferroelectric polarization will appear, but no further surface reconstruction is kinetically allowed ( Supplementary Fig. 4 ). Following this process, the room temperature bulk ferroelectric polarization is estimated to be P (298 K)=0.875 P 0 from the Landau model. Fixing the internal ferroelectric polarization of the LiNbO 3 to be 0.875 P 0 and relaxing the two nearest surface layers of the ferroelectric to model the actual experimental deposition of the graphene to the unpassivated surface at 298 K results in a situation where the graphene is responsible for passivating the extra surface charge on the ferroelectric. The doping levels in graphene adjacent to this surface structure can be visually illustrated by calculating the charge redistribution of the model system as the oxide and graphene are brought together ( Supplementary Note 1 ). The graphene on the P + surface exhibits an increase in electron density (red) while the graphene on the P − surface exhibits a reduction in electron density (blue) ( Fig. 3e ). In this state, the Dirac cones of the graphene are shifted by –0.245 eV ( n -type) or +0.245 eV ( p -type) with respect to the Fermi energy of native graphene as a consequence of contact with the P + and P − surfaces, respectively ( Fig. 3f ). The resulting symmetrical charge densities of n -type and p -type graphene yield 6.75 × 10 12 electrons cm −2 and 6.75 × 10 12 holes cm −2 , respectively, leading to a carrier density difference of 1.35 × 10 13 cm −2 ( Supplementary Fig. 5 ; Supplementary Note 2 ). We note that further testing of the induced charge densities reveals that sampling with a significantly higher k -point sampling shows the carrier densities to converge to ~5.0 × 10 12 carriers cm −2 , but with the same general behaviour. Regardless, this represents the maximum theoretical carrier density difference possible in this system, which is further reduced due to extrinsic effects arising from the combination of exposure to air and water during the graphene transfer process. Given the deviation of the estimated experimental carrier density values from this upper limit, we propose a defect-mediated carrier density reduction in graphene. Experimentally, the average defect density in the graphene on LiNbO 3 can be extracted by averaging the Raman spectra for all dark or bright stripes ( Fig. 1 ), which indeed yields an integrated D/G intensity ratio of ~7%, indicating generally low but non-negligible defect density. Locally, however, the defect concentration maybe higher as shown in the spatially resolved D/G intensity ratio ( Supplementary Fig. 6 ). At our ambient oxidizing conditions, graphene could accumulate O-species defects (adatoms) through its reaction with O 2 and H 2 O, leading to epoxides and/or hydroxyls [37] as well as chemisorbed and/or physisorbed O 2 molecules [38] ( Supplementary Fig. 7 ). The thermodynamics of formation of these defects on free-standing graphene and on graphene in close contact to LiNbO 3 reveals that the LiNbO 3 substrate enhances the stability of chemisorbed defects on graphene, leading to favourable epoxidation and hydrolyxation on the graphene/ P + and graphene/ P − surfaces, respectively ( Supplementary Fig. 8 ). For each case, the defect leads to a local carrier redistribution ( Supplementary Figs 9 and 10 ; Supplementary Note 3 ). Quantitatively, we examine epoxide and hydroxyl groups at the graphene/ P + LiNbO 3 and graphene/ P − LiNbO 3 interfaces, respectively. Physisorption of O 2 molecules on the graphene vacuum surface of both the P + and P − sides of the LiNbO 3 is discussed ( Supplementary Fig. 11 ). The epoxide and hydroxyl groups react with the surface Li + ions and form Li–O bonds. These chemical reactions with the LiNbO 3 surface lead to severe consequences on the electronic structure for the high defect concentration simulations completed herein (that is, 1 defect per every 8 graphene unit cells, which is limited by the size of the supercell we can utilize). In the epoxide on graphene/ P + LiNbO 3 case, the highly localized interactions lead to a gap opening with partially occupied localized defect states near the conduction band edge. This, in turn, inhibits graphene from possessing the n -type character while enhancing the p -type character on the defect-free graphene/ P − LiNbO 3 surface ( Fig. 4c ). In the hydroxyl on graphene/ P − LiNbO 3 case, the OH dissociates when the proton binds to a surface O, leading to a similar gap opening in the graphene with partially occupied gap states coming from the defects ( Fig. 4d ). The graphene facing the P + surface of LiNbO 3 , on the other hand, maintains its n -type character. We expect a less severe electronic structure change for lower defect concentration (that is, there would not be a gap opening). In general, O-species transforming sp 2 -type carbon orbitals into sp 3 -type lead to a reduction of mobile carrier density that decays over distance with Friedel oscillations ( Supplementary Fig. 10 ). As shown for the epoxide-type defect, the mobile carrier density can be reduced by as much as 2 × 10 12 cm −2 for a defect density of 1 defect per every 32 graphene unit cells. 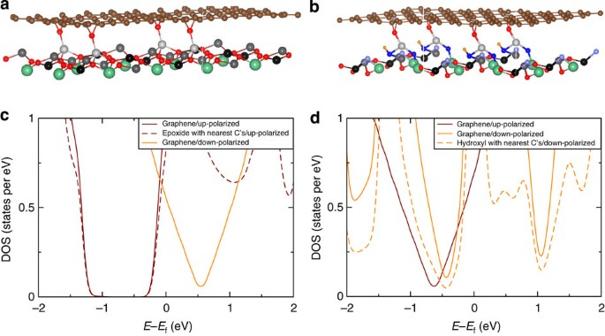Figure 4:Interfacial chemistry of the defective graphene/LiNbO3(0001) interface. (a) The atomic structure of the graphene and the top layer of the up-polarized LiNbO3surface with an epoxide at the interface (seeFig. 3cfor legend). (b) The atomic structure of the graphene and the top layer of the down-polarized LiNbO3surface with a hydroxyl at the interface (seeFig. 3cfor legend; additionally, the small orange spheres represent the hydrogen atoms). (c) The electronic structure of the graphene sheets and defect for the structure shown ina, demonstrating a gap opening on the graphene/up-polarized due to the interaction with the epoxide defect. This yields a relatively lower carrier concentration for the graphene on theP+surface (electrons) as compared to the one on theP−surface (holes). (d) The electronic structure of the graphene sheets and defect for the structure inb, illustrating gap opening with gap defect states in the graphene/down-polarized due to the reaction with the hydroxyl defect. The graphene on theP+remainsn-type. Incandd, projections of the defect plus nearest neighbour carbons are shown as dash lines; these states are highly localized charges as suggested inSupplementary Figs 9and10. Figure 4: Interfacial chemistry of the defective graphene/LiNbO 3 (0001) interface. ( a ) The atomic structure of the graphene and the top layer of the up-polarized LiNbO 3 surface with an epoxide at the interface (see Fig. 3c for legend). ( b ) The atomic structure of the graphene and the top layer of the down-polarized LiNbO 3 surface with a hydroxyl at the interface (see Fig. 3c for legend; additionally, the small orange spheres represent the hydrogen atoms). ( c ) The electronic structure of the graphene sheets and defect for the structure shown in a , demonstrating a gap opening on the graphene/up-polarized due to the interaction with the epoxide defect. This yields a relatively lower carrier concentration for the graphene on the P + surface (electrons) as compared to the one on the P − surface (holes). ( d ) The electronic structure of the graphene sheets and defect for the structure in b , illustrating gap opening with gap defect states in the graphene/down-polarized due to the reaction with the hydroxyl defect. The graphene on the P + remains n -type. In c and d , projections of the defect plus nearest neighbour carbons are shown as dash lines; these states are highly localized charges as suggested in Supplementary Figs 9 and 10 . Full size image The collective effect of the defects studied here is therefore responsible for the intrinsic behaviour of the graphene on the P + surface of LiNbO 3 and the lower than expected hole concentration when coupled to the P − surface of LiNbO 3 in devices at ambient conditions. Thus the electrons and holes necessary for polarization charge screening that are expected to reside in the graphene are, as observed in the experiments in this study as well as in previous reports, reduced due to the disruption in the mobile carrier density of graphene by the defects and the interaction of these with the underlying oxide substrate. Ultimately, these unique results provide important insights into the complexity and limitations of producing these couples between dissimilar materials, and provide guidance on what would be required to maximize coupling between ferroelectric polarization and charge carriers in graphene. In the end, the induced carrier density difference in graphene on different polarities of ferroelectric domains can only be fully understood when one considers the interfacial-chemistry-moderated consequence of the ferroelectric polarization in LiNbO 3 surfaces. Photocurrent in ferroelectrically defined p – n junctions Having established the nature of and mechanism for the carrier differences observed in the graphene/ferroelectric couples, we now consider the exploitation of the observed doping mechanisms for future devices based on the creation of spatially defined p–n junctions in graphene. In addition to the creation of spatially periodic doping regimes, the experimentally observed Dirac point voltage difference between graphene on up- and down-polarized LiNbO 3 ( Fig. 2d ) also clearly demonstrates that the application of top-gate voltages allows for a shift from p – i to p – n junctions. For the particular device shown here, a voltage between 0.1 and 0.3 V induces n -type behaviour in regions on up-polarized domains, while the graphene on down-polarized domains remains p -type. Thus, p–n junctions can be turned on or off through the application of a single gate voltage to the entire channel area, extending the capability of localized carrier density modulations to periodic carrier type variations. To demonstrate the existence of p–n junctions in graphene/ferroelectric hybrid structures, we measured spatially resolved photocurrent. In this experimental set-up, a laser with a small spot size is scanned across a graphene device with grounded electrodes. The induced photocurrent is measured at one of these contacts. At local potential steps, the internal electric field and photothermoelectric currents due to the carrier density and type-dependent Seebeck coefficient cause excited carriers in the graphene to be separated and accelerated into opposite directions [39] , [40] . The remarkable capability of the graphene/ferroelectric hybrid structures to create p–n junctions at the ferroelectric domain walls through the application of a single gate potential becomes apparent in the photocurrent response of top-gated graphene devices on periodically poled LiNbO 3 ( Fig. 5 ). Application of a single gate voltage (0.4 V for this device) shifts the potential landscape exhibited by the polarization to create a p – n junction between two adjacent domains. A maximum photocurrent response appears near the domain wall position (independently determined by the LiNbO 3 E (TO8) Raman peak frequency shift). On the basis of the spatially resolved photocurrent response, a schematic band diagram can be constructed ( Fig. 5 ), which corresponds well to our theoretical predictions. The p – n junction at the domain wall results in the maximum photocurrent, while the smaller band bending at the electrode edges, which is caused by the p -doping of graphene close to or underneath the metal contacts [41] , [42] , results in a moderate response. The different photocurrent magnitudes at the edges indicate that the chosen gate voltage results in different amounts of band bending at the two contacts. The magnitude of the photocurrent obtained for this device is of the expected order of magnitude for the observed carrier density difference ( Supplementary Note 4 ). The qualitative agreement of the photoresponse of the graphene/ferroelectric hybrid structure with results obtained utilizing split-gate configurations [40] , [43] underscores the importance of simplified creation and control of p – n junctions by placing graphene on polydomain ferroelectrics. 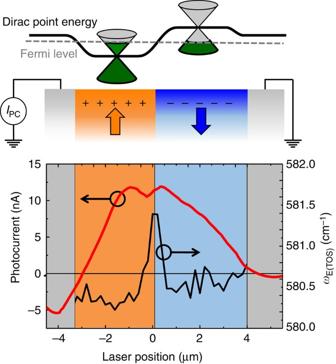Figure 5:Photocurrent response of a ferroelectricity-inducedp–njunction in graphene. The red line represents the photocurrent response of a top-gated graphene transistor with a gate voltage of 400 mV on periodically poled LiNbO3. The simultaneously detected RamanE(TO8) frequency (black) along the same line was used to identify the down-polarized (blue) and up-polarized (orange) domains of the LiNbO3. Grey shading corresponds to the Ti/Pd contacts. A schematic band diagram can be constructed based on the experimental observations. Figure 5: Photocurrent response of a ferroelectricity-induced p–n junction in graphene. The red line represents the photocurrent response of a top-gated graphene transistor with a gate voltage of 400 mV on periodically poled LiNbO 3 . The simultaneously detected Raman E (TO8) frequency (black) along the same line was used to identify the down-polarized (blue) and up-polarized (orange) domains of the LiNbO 3 . Grey shading corresponds to the Ti/Pd contacts. A schematic band diagram can be constructed based on the experimental observations. Full size image In conclusion, we have demonstrated spatially defined carrier density and type modulations in graphene arising from the Kronig–Penney potential landscape induced by an underlying periodically poled ferroelectric. Utilizing new insights about the graphene/ferroelectric interface obtained from DFT calculations, as well as scanning Raman spectroscopy and photocurrent imaging, we have shown that the polarization direction of a ferroelectric oxide can control the carrier density in graphene. While n - and p -doping of graphene on the up- and down-polarized surfaces is expected from an intuitive picture, detailed theoretical studies on the influence of surface reconstructions, polar stacking, temperature-dependent polarization and O-derived defects in the graphene have shown the importance of the interface in moderating the doping effect of the ferroelectric polarization. In a realistic device in air, the influence of adsorbed defects leads to an overall offset towards p -doping observed in the experimental carrier densities on different domains, which is explained by the DFT calculations of the model system with defects leading to carrier reduction. The resulting potential steps at the ferroelectric domain walls are comparable to results obtained with split-gate geometries, and lead to an array of spatially periodic p – i junctions in graphene exposed to an ambient environment, which can be continuously tuned from p + – p to n – n + junctions through the application of a single global gate potential. Although beyond the scope of this work, approaches combining nanoscale, deterministic domain engineering and top-gating could enable the study and the use of a relativistic phenomena based on chiral properties of electrons and holes in graphene. Such an approach could represent a new direction for developing advanced capabilities required for next-generation nanoelectronic and optoelectronic devices. Graphene growth and transfer Single-layer graphene with low defect density was grown on ultra-pure Cu foils (Alfa Aesar 10950). After annealing in 300 mtorr hydrogen atmosphere (flow rate 7 cm 3 min −1 ) at 1,000 °C for 30 min, a flow of 60 cm 3 min −1 of CH 4 was introduced for 20 min in a quartz tube containing the Cu foil. After cooling rapidly to room temperature with both gases flowing, the resulting graphene samples were transferred to thoroughly cleaned single crystals of LiNbO 3 using a one-touch wet-transfer method [15] . Raman studies Two-dimensional Raman maps and atomic force microscopy images of the same area were acquired with a WITec Confocal Raman Microscope alpha300. Gate-dependent Raman experiments and photocurrent microscopy were performed on a Jobin Yvon Labram HR800 micro-Raman spectrometer integrated with an Agilent Semiconductor Parameter Analyzer 4155 C. In all cases, 532 nm laser excitation and 100 × air objectives (laser spot size ) were used. The laser intensity was kept below or around 1 mW to ensure that laser-induced heating does not introduce artefacts. All peaks were fitted with a single Lorentzian. For the average spectra of dark and bright stripes in Fig. 1c , the point spectra acquired in each stripe were averaged and then fitted to a single Lorentzian. For gate-dependent measurements, a single line scan across multiple domains was used and the peak position results were averaged. Device fabrication and characterization Transistor devices were fabricated via electron beam evaporation of Ti/Pd source and drain electrodes with polymer electrolyte top gates prepared through the dissolution of LiClO 4 .3H 2 O and poly(ethylene oxide) (Sigma Aldrich, weight average molecular weight=100,000) in acetonitrile with 2.4:1:10 polymer to salt to solvent weight ratios similar to ref. 31 . The electrolyte solution was spin-coated onto the graphene devices at 3,000 r.p.m. for 30 s. Utilizing the Debye length with the dielectric permittivity , the thermal energy and the electrolyte concentration ρ =2.4 mol l −1 , the gate capacitance can be estimated to be C g = ε 0 ε r / λ =4 μF cm −2 . The carrier concentration can then be calculated using equation (1) from ref. 24 : utilizing ν F =1 × 10 6 m s −1 as the Fermi velocity in graphene [1] . Density functional theory First-principles calculations with a plane-wave basis set were performed using the local density approximation (LDA) [44] , as implemented in the QUANTUM ESPRESSO [45] code. Test calculations were also performed with the generalized gradient approximation and the van der Waals density functional yielding to similar electronic properties as LDA results. All atoms were represented by norm-conserving, optimized [46] , designed nonlocal [47] pseudopotentials generated using the OPIUM package. All the calculations employed a 50-Ry plane-wave energy cutoff. Atoms within two unit cells from the interface were allowed to relax while the rest of the slab was fixed to bulk atomic positions, simulating a range of different ferroelectric polarizations. The atoms were relaxed until the forces were <10 meV Å −1 . For the 2 × 1 surface reconstruction relaxation, the Brillouin zone was sampled with 6 × 12 × 1 Monkhorst-Pack k -point grids [48] explicitly including the Γ, K and M high-symmetry points. For high quality and well-converged electronic structure calculations for the 2 × 1 surface ground state, the Brillouin zone was sampled with 30 × 60 × 1 k -point grids, the highest density computationally accessible to compute the density of states (DOS) of the graphene in the hybrid structure. Detailed tests on pristine graphene showed that this grid can overestimate the carrier density by a factor of 1.35. The slab structure used to model the graphene/ferroelectric interfaces contained 11 trilayers of ferroelectric LiNbO 3 with 2 × 1 (0001) surface cells and graphene 4 × 2 surface supercells on both sides of the slab. The in-plane LDA-optimized lattice constant of graphene was found to be 2.445 Å, in agreement with previous work [49] . This induces a lattice parameter mismatch of 2.7%, placing the graphene under tension. The slab structures are separated with >13 Å of vacuum, and the dipole correction [50] was added to remove the spurious interaction between different supercells. For the defect states, four (4 × 4) graphene supercells with: (1) an epoxide, (2) a pair of hydroxyls at the ortho position, (3) chemisorbed O 2 molecule and (4) physisorbed O 2 molecule were calculated. Hybrid structures of graphene/LiNbO 3 interfaces with O-species defects on either or both sides of the graphene were also calculated with the same computational parameters described above. How to cite this article: Baeumer, C. et al . Ferroelectrically driven spatial carrier density modulation in graphene. Nat. Commun. 6:6136 doi: 10.1038/ncomms7136 (2015).